Ultra-wide bandgap semiconductor Ga2O3power diodes Ultra-wide bandgap semiconductor Ga 2 O 3 based electronic devices are expected to perform beyond wide bandgap counterparts GaN and SiC. However, the reported power figure-of-merit hardly can exceed, which is far below the projected Ga 2 O 3 material limit. Major obstacles are high breakdown voltage requires low doping material and PN junction termination, contradicting with low specific on-resistance and simultaneous achieving of n- and p-type doping, respectively. In this work, we demonstrate that Ga 2 O 3 heterojunction PN diodes can overcome above challenges. By implementing the holes injection in the Ga 2 O 3 , bipolar transport can induce conductivity modulation and low resistance in a low doping Ga 2 O 3 material. Therefore, breakdown voltage of 8.32 kV, specific on-resistance of 5.24 mΩ ⋅ cm 2 , power figure-of-merit of 13.2 GW/cm 2 , and turn-on voltage of 1.8 V are achieved. The power figure-of-merit value surpasses the 1-D unipolar limit of GaN and SiC. Those Ga 2 O 3 power diodes demonstrate their great potential for next-generation power electronics applications. Advanced semiconductor material holds great promise of providing higher conversion efficiency as well as maintaining higher voltage for modern industrial- and consumer-scale power electronics. Ultra-wide bandgap (UWB) semiconductor with general bandgap ( E g ) greater than 4 eV can sustain a higher critical field ( E c ) and hence a higher blocking voltage is achievable at a smaller resistance and power electronic component dimension, which turns out to be more efficient than its narrow bandgap material Si and wide bandgap material GaN and SiC counterparts, as summarized in Table 1 of Supplementary Information. The general concept lies behind is that the high electric-field ( E ) and high temperature driven of the electron excitation from valance band to conduction band is inherently suppressed by the UWB. Therefore, power electronics based on UWB materials are spontaneously endowed with high breakdown voltage (BV) at a lower material thickness and resistance. Combined with good mobility ( μ ), a crucial power device parameter Baliga’s figure-of-merit (B-FOM~ μ × E c 3 ) of UWB semiconductors could be several or tens of folds of those wide bandgap materials GaN and SiC as well as more than thousands of times of narrow bandgap material Si [1] , [2] . However, it should be noted that the major tyranny of the UWB forbids achieving effective both n- and p-type doping simultaneously. Among those intriguing UWB semiconductor materials, the emerging Ga 2 O 3 is now regarded as one of the most promising materials for next-generation high-power and high-efficiency electronics, due to its cost-effective melt-grown large-scale and low defect density substrate as well as the controllable n-type doping [3] . Ga 2 O 3 with E g = 4.6–4.8 eV, high E C = 8 MV/cm and decent intrinsic μ = 250 cm 2 /Vs has yielded a B-FOM to be around 3000, which is four times GaN and ten times SiC. Being the mainstream of the UWB semiconductor, Ga 2 O 3 -based power electronics are expected to bring higher blocking voltage at a lower specific on-resistance ( R on,sp ) for power switching applications. Tremendous efforts have been dedicated to explore the material property and push the device limit, and hence significant progresses are acquired during the past 5 years. Despite those intriguing achievements, it should be noted that those performances especially the representative device parameter power figure-of-merit (P-FOM = BV 2 / R on,sp ) are much inferior to the projected material limit, or even cannot be comparable with the 1-D unipolar limit of the GaN and SiC [4] , [5] . Like other UWB semiconductors with the difficulties of achieving both highly conductive p- and n-type materials at the meantime, one of the major obstacles is the lack of p-type Ga 2 O 3 which can be utilized as the PN homo-junction termination for the BV improvement. It was calculated that shallow acceptor does not exist and it was also predicted that the holes are self-trapped inherently [6] . As a result, unipolar Ga 2 O 3 power electronics dominate most of the research and few reports are available about the bipolar transport study. Due to the challenge of realizing p-type Ga 2 O 3 on lightly-doped n-type Ga 2 O 3 layer, the BV of the vertical Ga 2 O 3 power diodes was limited, although various types of edge termination (ET) methods were employed [7] . On the other hand, some wide-bandgap p-type materials like NiO x with E g of 3.8–4 eV and Cu 2 O with E g ~ 3 eV, controllable doping and decent hole mobility of 0.5–5 cm 2 /V s turn out to be a good counterpart of p-type Ga 2 O 3 to boost the diodes performance [8] , [9] . The combination of p-NiO x and n-Ga 2 O 3 is a feasible route for the Ga 2 O 3 development, and the recent progress of the Ga 2 O 3 PN hetero-junction (HJ) diodes shows a P-FOM of 1.37 GW/cm 2 , which is comparable to the P-FOM value of state-of-the-art Schottky barrier diodes (SBDs) [10] , [11] . Even incorporating p-NiO x into Ga 2 O 3 material system, the potential of Ga 2 O 3 HJ PN diodes is only explored for less than 10% of the material limitation. Meanwhile, the conductivity modulation effect is observed in Ga 2 O 3 HJ PN diodes, indicating the holes can be injected in the Ga 2 O 3 layer [12] . However, under what bias condition and to what extent the conductivity modulation can impact the R on,sp are still not explored. In addition, the in-depth understanding of bipolar transport in the Ga 2 O 3 layer, especially hole transport and lifetime extraction are still forfeiting. Against the generally believed holes are self-trapped, the hole lifetime is a crucial and fundamental parameter to determine whether the bipolar transport is about to happen and to what extent it will impact the PN diode performances. Another critical issue regards the practical application of UWB PN diode is the requirement of low turn-on voltage ( V on ) for high-efficiency application, since the general forward bias ( V F ) is limited to be around 3 V. This is very challenging for homo-junction PN diode for wide bandgap semiconductor GaN and SiC with V on ~ 3 V, regardless of the even wider bandgap Ga 2 O 3 . In this article, a general design strategy of UWB semiconductor power diodes is provided to achieve high BV and low R on,sp simultaneously through the introduction of hole injection and transport in Ga 2 O 3 to minimize the R on,sp , suppressing the background carrier density to improve the BV, employing low conduction band offset p-NiO x to reduce V on , and a composite E management technique with implanted ET and field plate architecture to further strengthen the BV. We setup a milestone of the UWB power diodes by acquiring a BV of 8.32 kV and P-FOM = BV 2 / R on,sp of 13.21 GW/cm 2 , which is a record P-FOM value among all types of UWB power diodes to date, and it also exceeds the 1-D unipolar limit of GaN and SiC. Meanwhile, a conductivity modulation phenomenon induced bipolar transport of electron and hole pairs is identified with hole lifetime determined to be 5.4–23.1 ns. Considering some real application circumstances of diodes at a V F of 3 V, benchmarking of the BV and R on,sp extracted at V F = 3 V also shows a record P-FOM value to date, validating the great promise of UWB power diodes for next-generation high-voltage and high-power electronics. High BV and low R on,sp design strategy and implementation The most intriguing aspect of β-Ga 2 O 3 is that its native substrate can be substantially grown by the melt-grown methodology, which lays a basic foundation for low-cost and large-diameter with low defect density substrate [13] . The β-Ga 2 O 3 epi-layer can be epitaxied by various routes, such as molecular beam epitaxy, metalorganic chemical vapor deposition (MOCVD), mist-CVD, halide vapor phase epitaxy (HVPE), and some other low-cost techniques [14] , [15] . HVPE is the most widely adopted methodology for balancing the epitaxial speed, substrate size, defect density, and complicity. The β-Ga 2 O 3 background doping regulation is a challenge, resulting in a non-controllable electron density of 2–4 × 10 16 cm −3 . Unintentional doping from precursors like Si or H, and defects like O vacancies all contribute to the n-type conduction in the β-Ga 2 O 3 layer. Ideal power devices should embrace high BV and low R on,sp to provide high blocking capability and low loss simultaneously [16] . In order to improve the BV of the UWB Ga 2 O 3 power diodes, the minimal doping concentration is the first essential, since the slope of the E is governed by the doping concentration [16] . Summarized in Supplementary Fig. 1 , it was found that the BV of the reported Ga 2 O 3 power diodes is limited to be less than 3 kV, where the donor concentration is the major tyranny. Some other subsidiary factors like ETs or advanced E management techniques are all prerequisites for a minimized peak E at the anode edge to achieve a high desirable BV. PN junction is one of the most straightforward approaches to suppress the peak E at the interface. However, the forfeit of the p-Ga 2 O 3 on the n-Ga 2 O 3 makes the PN home-junction an impossible mission to further explore the maximum BV potentials of diodes. It should be noted that only extending the spacing of two electrodes to increase the BV is of marginal value by sacrificing the R on,sp and averaged E. In terms of manipulating the R on,sp , to increase the doping concentration seems to be the simplest, however, the BV will be essentially compromised. A unique physical phenomenon of power diode, which is called conductivity modulation of the PN or PIN junction at forward bias will substantially guarantee a low R on,sp even at a low doping concentration. Regardless of the challenge on the formation of PN homo-junction, the high V on > 4 V is another suffering for the Ga 2 O 3 homo-junction PN diodes. Recently, the implementation of the p-NiO x into the Ga 2 O 3 system opens up another route for expanding the Ga 2 O 3 application from the SBDs to the HJ PN diode [17] , [18] , [19] , [20] . Although the performance of the Ga 2 O 3 HJ diode is still inferior to the SBDs at current stage, however, we argue that some fundamental limitations which have haunted the Ga 2 O 3 power diodes research for a decade could be essentially clarified. First, p-NiO x flavors a low conduction band offset of ~2.1 eV such that the high V on issue of the homo-junction could be partially resolved. Second, with a PN HJ structure, the conductivity modulation is theoretically expected so that the R on,sp can be minimized at a low doping concentration and high V F . In addition, by combining the ETs and advanced E management, the BV can be further enhanced. Comparison of the E management strategies is summarized in Supplementary Fig. 2 . 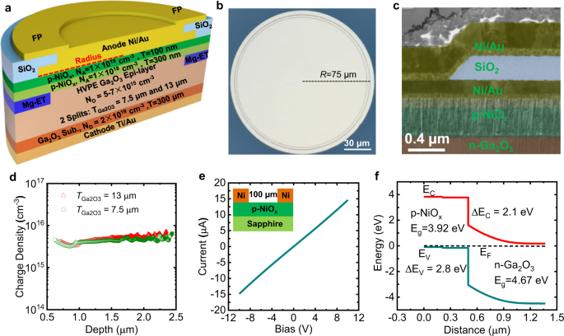Fig. 1: UWB power diodes design and implementation. a3-D cross-sectional schematic of the Ga2O3power diodes with HJ architecture and composite electric field management.bTop view of a fabricated Ga2O3power diode.cFalse-colored SEM image of the cross-sectional anode field plate region with p-NiOxthickness of 400 nm.dExtracted carrier concentration of two representative samples with concentration of 5 × 1015−7 × 1015cm−3.eCurrent-voltage behavior of the Ni pads on p-NiOxwithNA= 1019cm−3, showing an Ohmic contact.fSimulated band diagram of the p-NiOx/n-Ga2O3HJ structure. The band bending occurs in n-Ga2O3and the conduction band offset is only 2.1 eV, showing the great promise of lowVoneven for a UWB material. Figure 1a shows the 3-D cross-sectional image of two representative Ga 2 O 3 HJ PN diodes, the top view image is exhibited as Fig. 1b , and the false-colored scanning electron microscopy (SEM) image at the crucial area of the anode edge is listed in Fig. 1c . In the Ga 2 O 3 power diodes, the doping concentration of the Ga 2 O 3 epi-layer is suppressed from the 2 × 10 16 cm −3 to around 5–7 × 10 15 cm −3 for two wafers with different thicknesses by adopting a long duration of the oxygen thermal anneal process, as shown in Fig. 1d [21] . C – V curves are shown in Supplementary Fig. 3 . Heavily doped p-NiO x layer on top is utilized to form an Ohmic contact, as described in Fig. 1e . The simulated energy band diagram of the p-NiO x / n -Ga 2 O 3 HJ is shown in Fig. 1f with the conduction band and valance band offset to be 2.15 eV and 2.8 eV, respectively. The ET process by Mg doping to form a high-resistivity region underneath the electrode is utilized to withstand a high E and the coupled field plate is implemented to further mitigate crowded peak E at the anode edge [15] . Fig. 1: UWB power diodes design and implementation. a 3-D cross-sectional schematic of the Ga 2 O 3 power diodes with HJ architecture and composite electric field management. b Top view of a fabricated Ga 2 O 3 power diode. c False-colored SEM image of the cross-sectional anode field plate region with p-NiO x thickness of 400 nm. d Extracted carrier concentration of two representative samples with concentration of 5 × 10 15 −7 × 10 15 cm −3 . e Current-voltage behavior of the Ni pads on p-NiO x with N A = 10 19 cm −3 , showing an Ohmic contact. f Simulated band diagram of the p-NiO x /n-Ga 2 O 3 HJ structure. The band bending occurs in n-Ga 2 O 3 and the conduction band offset is only 2.1 eV, showing the great promise of low V on even for a UWB material. 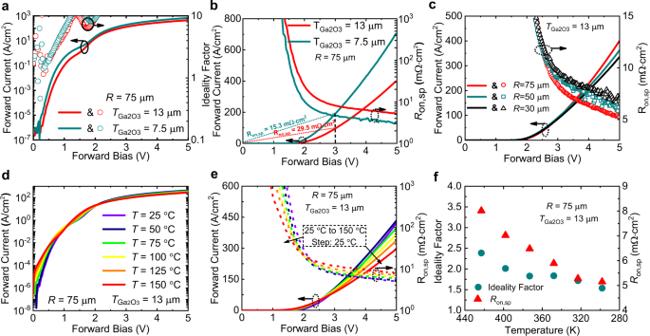Fig. 2: UWB Ga2O3power diodes forward characteristics. aForward current-voltage-ideality factor characteristics of two Ga2O3power diodes withTGa2O3= 7.5 and 13 μm.bForward current–voltage-specific on-resistanceRon,spcharacteristics of the same diodes asa. A decentVon= 1.8 V with minimal Diff.Ron,sp= 2.9 and 5.24 mΩ cm2as well as extracted overallRon,sp(@VF= 3 V) of 15.3 and 29.5 mΩ cm2forTGa2O3= 7.5 and 13 μm are achieved.cRadius-dependent forward current-voltage-resistance curves for diodes withTGa2O3= 13 μm. T-dependentdlog-scale andelinear-scale forward characteristics of diode withTGa2O3= 13 μm. On/Off ratio of 1010and 108are achieved forT= 25 °C and 150 °C, respectively. At all temperatures,Ron,spdrops whenVFincreases, verifying the conductivity modulation effect.fExtracted T-dependent ideality factor andRon,spvalues ase. Full size image Diodes characterizations Figure 2a compares the log-scale forward current-forward bias-ideality factor ( I F - V F - η ) characteristics of two Ga 2 O 3 HJ PN diodes with Ga 2 O 3 thickness (T Ga2O3 ) of 7.5 and 13 μm at a radius of 75 μm. The kink effect observed at V F around 1.5 V is related to the variation of the barrier height and ideality factor, which is most likely to be induced by the two different barriers connected in parallel. I F on/off ratio of 10 9 −10 10 and η smaller than 2 can last for 4–5 decades of the I F . Figure 2b shows the linear-scale forward I F - V F - R on,sp curves of the same diodes as Fig. 2a . Even with a PN HJ structure, a relatively decent V on = 1.8 V is acquired, which is much smaller than the V on of SiC and GaN PN diodes. The small V on is benefited from two aspects, the small conduction band offset between p-NiO x and n-Ga 2 O 3 and the interface recombination current [17] . Minimal Diff. R on,sp is extracted to be 2.9 and 5.24 mΩ cm 2 for T Ga2O3 = 7.5 and 13 μm, respectively. Unlike SBDs with increased R on,sp at an increased V F , the R on,sp of the Ga 2 O 3 HJ PN diodes drops at an increased V F , most likely due to bipolar transport-induced conductivity modulation effect. It should be noted that such conductivity modulation effect is the key to enable the simultaneous achievement of low R on,sp and high BV. Figure 2c describes the radius-dependent I F - V F - R on,sp curves for diodes with T Ga2O3 = 13 μm. Log-scale I F - V F characteristic is summarized in Supplementary Fig. 4 . By increasing the radius, the insulating Mg implanted region constitutes to a smaller portion of the area so that R on,sp decreases when radius increases. The resistance (Res.) contribution from each layer based on the equation Res. = thickness/( N D × μ × q ) is summarized in Supplementary Fig. 5 [22] . For diodes with T Ga2O3 = 7.5/13 μm, N D = 6 × 10 15 cm −3 , μ = 200 cm 2 /Vs, and q = 1.6 × 10 −19 C, the resistance of the drift layer is calculated to be 3.89/6.77 mΩ cm 2 . It should be noted that this calculation is based on the low-level injection prerequisite. At V F = 5 V, conductivity modulation effect of the HJ PN diode begins to dominate so that the R on,sp drops, which is favorable for resistance minimization. Figure 2 d and  e summarizes the T-dependent linear-scale I - V - R on,sp and log-scale I F - V F of the diode with radius = 75 μm and T Ga2O3 = 13 μm. On/off ratios of 10 10 and 10 8 are achieved at T = 25 °C and 150 °C, respectively. At all temperature ranges, the differential (Diff.) R on,sp drops at an increased V F , verifying the conductivity modulation effect of the Ga 2 O 3 HJ PN diodes. Figure 2f shows the extracted T-dependent ideality factor η and R on,sp from temperatures of 25–150 °C. The η is extracted from the forward current equation J = J s (exp( qV F / ηkT ) − 1), whereas J s is the reverse saturation current, V F is the applied forward bias, q is the electron charge, k is the Boltzmann’s constant, and T is the absolute temperature. The η is extracted to be around 1.5 at T = 25 °C. Fig. 2: UWB Ga 2 O 3 power diodes forward characteristics. a Forward current-voltage-ideality factor characteristics of two Ga 2 O 3 power diodes with T Ga2O3 = 7.5 and 13 μm. b Forward current–voltage-specific on-resistance R on,sp characteristics of the same diodes as a . A decent V on = 1.8 V with minimal Diff. R on,sp = 2.9 and 5.24 mΩ cm 2 as well as extracted overall R on,sp (@ V F = 3 V) of 15.3 and 29.5 mΩ cm 2 for T Ga2O3 = 7.5 and 13 μm are achieved. c Radius-dependent forward current-voltage-resistance curves for diodes with T Ga2O3 = 13 μm. T-dependent d log-scale and e linear-scale forward characteristics of diode with T Ga2O3 = 13 μm. On/Off ratio of 10 10 and 10 8 are achieved for T = 25 °C and 150 °C, respectively. At all temperatures, R on,sp drops when V F increases, verifying the conductivity modulation effect. f Extracted T-dependent ideality factor and R on,sp values as e . Full size image Based on the simulation, it is very interesting to find that hole concentration in the Ga 2 O 3 layer at the HJ-interface is comparable with the Ga 2 O 3 doping concentration of 6 × 10 15 cm −3 at V F = 3.5 V, as shown in Supplementary Figs. 6 and 7 . That is to say, the hole injection-related conductivity modulation can help to reduce the R on,sp only with V F ≥ 3.5 V, since the hole is with more than 1 order of magnitude lower mobility. The simulation result is in good agreement with the forward I F – V F characteristic, since the R on,sp = 7 mΩ cm 2 (at V F = 3.5 V) roughly equals to the resistance summary of p-side Ohmic contact, p-NiO x layer, n-Ga 2 O 3 drift layer, n + -Ga 2 O 3 substrate and n-side Ohmic contact. In other words, the hole injection and conductivity modulation are negligible at the V F range of V on = 1.8 V to 3.5 V, due to significant valance band offset between p-NiO x and n-Ga 2 O 3 , so that few holes can be injected across this barrier. At V F ~ 3.5 V, holes are injected from p-NiO x to n-Ga 2 O 3 most likely via trap assisted tunneling and hopping mechanisms. By increasing the V F beyond 3.5 V to lower the PN HJ barrier, more holes are injected into n-Ga 2 O 3 layer and hence high level injection phenomenon will raise the electron concentration in the Ga 2 O 3 layer to maintain the charge neutrality condition. Therefore, the R on,sp is further reduced when the V F is increased. At V F = 5 V, the hole concentration is simulated to be 3.8 × 10 16 cm −3 and 6 × 10 15 cm −3 at HJ-interface and 6 μm away from the HJ-interface, respectively. The averaged hole (also electron) concentration is extracted to be 1.9 × 10 16 cm −3 within this 6-μm range, by integrating concentration and then divided by the total length of 6 μm. Therefore, the resistance of the significant hole injection region is roughly calculated to be 1.32 mΩ cm 2 , by considering the electron mobility of 150 cm 2 /Vs at this electron concentration. By adding up another 7-μm low level injected Ga 2 O 3 layer resistance of 6.77/13 × 7 = 3.65 mΩ cm 2 , the 13-μm Ga 2 O 3 drift layer owns a R on,sp of 4.97 mΩ cm 2 . This estimation of the R on,sp coincides with our extracted R on,sp from the I F – V F , verifying the correctness of the explanation, hole concentration simulation, and calculation of the hole injection into the Ga 2 O 3 layer. The T-dependent reverse I – V characteristics of diode with T Ga2O3 = 7.5 μm are plotted in Fig. 3a from T = 25–150 °C. By increasing the T , I R increases, indicating a non-avalanche breakdown behavior. Even at T = 150 °C, the I R is just 1 mA/cm 2 at a reverse bias of 3 kV. By further pushing the reverse bias to 5.1 kV we observe a hard breakdown with T Ga2O3 = 7.5 μm, as indicated in Fig. 3b . The averaged E field is calculated to be around 6.45 MV/cm by considering E = 5.1 kV/(0.4 μm + 7.5 μm). Combined with the R on,sp = 2.9 mΩ cm 2 , the P-FOM = BV 2 / R on,sp is yielded to be 8.97 GW/cm 2 . As for the diode with T Ga2O3 = 13 μm, a maximum BV of 8.32 kV is acquired at an I R = 0.2 mA/cm 2 , as exhibited in Fig. 3c . The as-measured figure is shown in Supplementary Fig. 8 . This BV = 8.32 kV is the highest BV value among all Ga 2 O 3 power FETs and diodes to date. As a result, the P-FOM is calculated to be (8.32 kV) 2 /5.24 mΩ cm 2 = 13.21 GW/cm 2 . Besides the record P-FOM, this HJ PN diode also has a high averaged E = 8.32 kV/(0.4 μm + 13 μm) = 6.2 MV/cm. 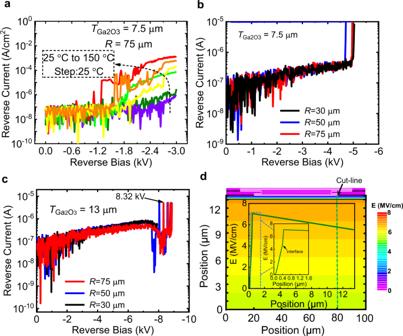Fig. 3: UWB Ga2O3power diodes with high breakdown voltages. aT-dependent reverse current–voltage characteristics of diode withTGa2O3= 7.5 μm. With increasedT,IRincreases, indicating a non-avalanche breakdown. Room temperature reverse current–voltage characteristics of diodes withTGa2O3= 7.5 μm (b) and 13 μm (c) at various radiuses. A BV of 5.1 kV and 8.32 kV are achieved for diodes withTGa2O3= 7.5 and 13 μm, yielding an averagedEof 6.45 MV/cm and 6.2 MV/cm, respectively.dSimulated E distribution of the diode with BV = 8.32 kV and TGa2O3= 13 μm. Due to the smallND= 6 × 1015cm−3, a fully depletion and a small E slope of the drift layer is observed. Figure 3d describes the E simulation result of the HJ PND with T Ga2O3 = 13 μm and BV = 8.32 kV. The simulated peak E in the p-NiO x layer is around 4.9 MV/cm, which is slightly lower than its theoretical limit, considering the 3.9 eV bandgap. The peak E at the p-NiO x side is lower when compared with the peak E at the Ga 2 O 3 side, due to much higher dielectric constant of p-NiO x . Due to the small N D and the depletion effect from the p-NiO x as well as the functionalities of the ET and coupled field plate, a fully depletion and small E slope are observed in the drift layer, resulting a peak E = 7 MV/cm in the Ga 2 O 3 at the HJ-interface. Fig. 3: UWB Ga 2 O 3 power diodes with high breakdown voltages. a T-dependent reverse current–voltage characteristics of diode with T Ga2O3 = 7.5 μm. With increased T , I R increases, indicating a non-avalanche breakdown. Room temperature reverse current–voltage characteristics of diodes with T Ga2O3 = 7.5 μm ( b ) and 13 μm ( c ) at various radiuses. A BV of 5.1 kV and 8.32 kV are achieved for diodes with T Ga2O3 = 7.5 and 13 μm, yielding an averaged E of 6.45 MV/cm and 6.2 MV/cm, respectively. d Simulated E distribution of the diode with BV = 8.32 kV and T Ga2O3 = 13 μm. Due to the small N D = 6 × 10 15 cm −3 , a fully depletion and a small E slope of the drift layer is observed. Full size image Holes in Ga 2 O 3 layer Similar to other UWB semiconductors like diamond, BN, and AlN, high ionization efficiency of n- and p-type doing simultaneously turns out to be a big challenge, considering the UWB nature of those UWB semiconductor materials. The direct observation of conductivity modulation is a straightforward evidence of bipolar transport and hole existence in the Ga 2 O 3 layer, which deviates from the general prediction that holes are less likely to occur in Ga 2 O 3 . Three reasons are attributed to the challenge of acquiring holes in Ga 2 O 3 , no calculated shallow acceptors, large effective mass from the flat valance band, and free holes tend to be self-trapped by polarons. However, we argue that with the unique PN HJ structure under high V F condition, holes from the heavily-doped p-NiO x are capable of being injected to the Ga 2 O 3 layer, although the hole mobility is relatively low. Under a very positive V F condition (e.g., 5 V), energy band of the p-NiO x is pulled down so that holes at the Fermi tail witness no significant barrier height to travel across the PN HJ-interface and then diffuse in the Ga 2 O 3 layer, leading to the conductivity modulation effect. In other words, the holes can be manufactured in the UWB Ga 2 O 3 layer by hole injection at a very positive V F . In order to verify the hole transportation and survival in the Ga 2 O 3 not so short by self-trapping effect of the polarons, hole lifetime extraction or measurement is urgently needed. The reverse recovery measurement technique is implemented to determine the hole lifetime in the Ga 2 O 3 layer, and the schematic of the measurements are summarized in Supplementary Fig. 9a [23] . Once the Ga 2 O 3 diode is switched from positive V F to a reverse bias, a period of time is needed to remove holes from the Ga 2 O 3 either via electron-hole pair recombination or to be trapped by polarons. The hole lifetime ( τ p ) can be determined by the equation τ p = t sd /(erf −1 ( I F /( I F + I R ))) 2 , whereas t sd , I F , and I R represent charge storage time, forward current, and reverse current, respectively [24] . During the reverse recovery measurement, the V F is extracted to be 2.97 V and 4.73 V for injection current of 5 mA and 25 mA, respectively, at a diode radius of 40 μm. Meanwhile, the subsequently applied reverse bias is −8 V. The reverse recovery and input–output measurement of the pulsed current–voltage characteristics of the UWB Ga 2 O 3 HJ PN diode at a diode current of 5 mA is shown in Fig. 4a . For the HJ PN diode, the I F is 5 mA which is 3 orders of magnitudes more than I R , so that I F /( I F + I R ) can be simplified to be 1. Then the τ p can be simplified to π /4 × t sd , which is ~80% of the t sd when the diode is switched until the anode current is recovered to be around 0. Therefore, hole lifetime τ p is determined to be 23.1 ns at a forward injection current I F of 5 mA. The τ p dependence on I F is summarized in Fig. 4b , with a minimal τ p of 5.4 ns. In order to exclude the subsidiary impact on the measurements, the reverse recovery measurement is performed on Ga 2 O 3 SBD (Supplementary Fig. 9b ) and the recovery time in the SBD is determined to be 1.8 ns, which is 1 order of magnitude lower when compared with the HJ PN diode. By injecting holes into the Ga 2 O 3 layer at high V F , the hole lifetime is then determined to be 5.4–23.1 ns. By combining the calculated hole effective mass ( m p *) of 4.46 m o (Supplementary Fig. 10 ), the hole mobility ( μ p ) can be roughly estimated by the equation μ p = q × τ p / m p *, yielding the μ p to be 1.93–8.3 cm 2 /Vs. Fig. 4: Hole lifetime determination in Ga 2 O 3 layer. a Time-dependent of the reverse recovery characteristics of Ga 2 O 3 HJ PN diode at a forward injection current of 5 mA. b Lifetime dependence on the forward injection current with current ranges from 5 mA to 25 mA. At current of 5 mA, the lifetime is determined to be 23.1 ns. At high V F condition, holes diffuse from p-NiO x to n-Ga 2 O 3 without seeing obvious barrier, so that the hole lifetime in the Ga 2 O 3 layer can be determined. Full size image Performance benchmarking The combination of the conductivity modulation induced low R on,sp and low doping concentration as well as the composite E regulation led record BV renders a substantial performance enhancement by setting a record P-FOM of all UWB power diodes (Fig. 5a ), including Ga 2 O 3 , diamond, and high Al-Al x Ga 1− x N ( x > 60%) power diodes [25] , [26] , [27] , [28] , [29] , [30] , [31] , [32] , [33] , [34] , [35] , [36] , [37] , [38] , [39] , [40] , [41] , [42] , [43] , [44] . Compared with all other Ga 2 O 3 power diodes, the BV of this work is around three times the previously reported best BV of 2.9 kV with a lower R on,sp . The most enticing aspect of this work is that the performance of the Ga 2 O 3 device exceeds the 1-D unipolar limit of the SiC and GaN. In terms of real application of the HJ PN diode in the circuit, the overall R on,sp at a general V F = 3 V instead of the minimal differential R on,sp is more realistic. In order to eliminate the impact of V on , an overall R on,sp of 15.3 mΩ cm 2 and 29.5 mΩ cm 2 are extracted for T Ga2O3 of 7.5 μm and 13 μm at a V F = 3 V, respectively, as shown in Fig. 2b . Benchmarking against all other state-of-the-art representative diodes, including SiC SBDs/JBS diodes/PN diodes and GaN SBDs/PN diodes with extracted R on,sp at a fixed V F = 3 V, our Ga 2 O 3 HJ PN diodes achieve a record of nowadays power diodes, as compared in Fig. 5b [33] , [45] , [46] , [47] , [48] , [49] , [50] , [51] , [52] , [53] . Even under the real application circumstance, the P-FOM = BV 2 / R on,sp of the Ga 2 O 3 power diodes still surpasses the 1-D unipolar limit of the SiC. These intriguing results verify the great promise of UWB semiconductor Ga 2 O 3 power diodes for next-generation high-voltage and high-power electronics. Fig. 5: Benchmarking UWB Ga 2 O 3 power diodes against state-of-the-art other diodes. a Minimal R on,sp versus BV of some representative UWB power diodes, including Ga 2 O 3 , diamond, and high-Al AlGaN, which are reported in the literatures. Our Ga 2 O 3 power diodes set a milestone for the UWB power diodes by breaking the 1-D unipolar figure-of-merit limit of GaN and SiC. b Extracted R on,sp (@3V) versus BV of some highest performance GaN, SiC, and diamond diodes. By considering some real application circumstances, the R on,sp = 3V/(I F @3 V) is preferred over the minimal R on,sp to eliminate the impact of the V on . GaN and SiC PN diodes are excluded due to the V on ~ 3 V. Our UWB power diodes demonstrate a substantial enhancement of the performance over other diodes by surpassing the 1-D unipolar limit of the SiC. The R on,sp extraction for lateral diodes is yielded by R on,sp = on-resistance × (anode–cathode spacing +1.5 μm transfer length for both electrodes). Full size image In summary, we show that UWB semiconductor Ga 2 O 3 power diodes are capable of delivering a record high BV 2 / R on,sp , which breaks the 1-D unipolar limit of the SiC and GaN figure-of-merit. The incorporation of suppressed background doping, HJ PN structure, and the composite electric field management technique yields a high BV which makes the averaged electric field approach the material limit. Taking advantage of the hole injection as well as the conductivity modulation, the R on,sp can be essentially minimized even the Ga 2 O 3 is with a low doping concentration. The hole lifetime is determined to be 5.4–23.1 ns, which verifies the existence of the hole in the Ga 2 O 3 layer. By carefully engineering the energy band offset, a decent V on can also be derived for a high efficiency rectifying. This unique technology by implementing the low doping material, electric field suppression, hole injection as well as the conductivity modulation, and energy band engineering offers an effective route for the innovation of other UWB power diodes, such as diamond, BN, high Al mole fraction Al x Ga 1-x N. Fabrication of UWB Ga 2 O 3 power diodes Ga 2 O 3 epi-wafers with epi-layer thicknesses of 7.5 μm and 13 μm were epitaxial by HVPE on a (001) substrate with substrate doping concentration of 2 × 10 19 cm −3 . Substrates were first thinned down from 650 μm to 300 μm by polishing to minimize on-resistance. Then, Ga 2 O 3 epi-wafers were annealed in the low-pressure-CVD furnace at 500 °C under the O 2 ambient to partially compensate the donors in the epi-layer. N-side Ohmic contacts were formed by evaporating Ti/Au metals followed with rapid thermal anneal at 450 °C. Angle-dependent Mg ion implantation was utilized to form a high-resistivity layer to serve as the ET. Bi-layers of p-NiO x were sputtered at room temperature with first and second layer doping concentration of 1 × 10 18 cm −3 and 1 × 10 19 cm −3 , respectively. 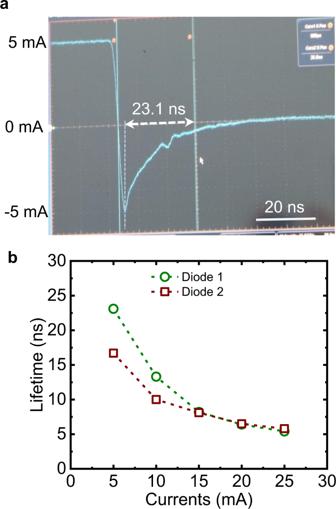Fig. 4: Hole lifetime determination in Ga2O3layer. aTime-dependent of the reverse recovery characteristics of Ga2O3HJ PN diode at a forward injection current of 5 mA.bLifetime dependence on the forward injection current with current ranges from 5 mA to 25 mA. At current of 5 mA, the lifetime is determined to be 23.1 ns. At highVFcondition, holes diffuse from p-NiOxto n-Ga2O3without seeing obvious barrier, so that the hole lifetime in the Ga2O3layer can be determined. 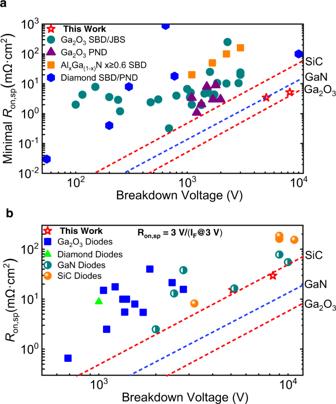Fig. 5: Benchmarking UWB Ga2O3power diodes against state-of-the-art other diodes. aMinimalRon,spversus BV of some representative UWB power diodes, including Ga2O3, diamond, and high-Al AlGaN, which are reported in the literatures. Our Ga2O3power diodes set a milestone for the UWB power diodes by breaking the 1-D unipolar figure-of-merit limit of GaN and SiC.bExtractedRon,sp(@3V) versus BV of some highest performance GaN, SiC, and diamond diodes. By considering some real application circumstances, theRon,sp= 3V/(IF@3 V) is preferred over the minimalRon,spto eliminate the impact of theVon. GaN and SiC PN diodes are excluded due to theVon~ 3 V. Our UWB power diodes demonstrate a substantial enhancement of the performance over other diodes by surpassing the 1-D unipolar limit of the SiC. TheRon,spextraction for lateral diodes is yielded byRon,sp= on-resistance × (anode–cathode spacing +1.5 μm transfer length for both electrodes). The doping concentration of the p-NiO x layer was confirmed by the Hall measurements and the Hall mobility of the second p-NiO x layer is 1.1 cm 2 /Vs. P-side Ohmic contacts were formed by depositing Ni/Au layers. The field plate was constructed by depositing 300 nm of SiO 2 , SiO 2 etching, and field plate metal evaporation. A summary of the device process schematic flow is shown in Supplementary Fig. 11 . Device characterizations The forward I – V and C – V characteristics were carried out by the Keithley 4200 semiconductor analyzer systems. Reverse I – V measurements were performed by Agilent B-1505A high voltage semiconductor analyzer systems with extended high-voltage module up to 10 kV. The hole lifetime measurements were carried out by reverse recovery measurement methods as Supplementary Fig. 9 .